Anchoring Cu1species over nanodiamond-graphene for semi-hydrogenation of acetylene The design of cheap, non-toxic, and earth-abundant transition metal catalysts for selective hydrogenation of alkynes remains a challenge in both industry and academia. Here, we report a new atomically dispersed copper (Cu) catalyst supported on a defective nanodiamond-graphene (ND@G), which exhibits excellent catalytic performance for the selective conversion of acetylene to ethylene, i.e., with high conversion (95%), high selectivity (98%), and good stability (for more than 60 h). The unique structural feature of the Cu atoms anchored over graphene through Cu-C bonds ensures the effective activation of acetylene and easy desorption of ethylene, which is the key for the outstanding activity and selectivity of the catalyst. Selectively hydrogenating remnant acetylene in the raw olefin streams to ethylene while avoiding the over-hydrogenation to undesired ethane is a key industrial reaction to manufacture polymer-grade raw materials for the production of polyethylene [1] , [2] , [3] . The most commonly used industrial catalyst for the reaction is based on supported Pd nanoparticles (NPs) modified by Ag additives [4] . Although the Pd-Ag catalyst prevents the usage of toxic promoters such as lead or sulfur (Lindlar catalyst) [5] , the extremely high cost of Pd leaves ample room for improving the cost-effectiveness in catalyst design. In an effort to develop environment-friendly and cost-effective catalysts, various approaches have been pursued, including (i) reducing the amount of noble metals by “site-isolation” strategy or engineering a minimal ensemble [6] , [7] , [8] , [9] , [10] , [11] and (ii) developing non-noble metals/metal oxides catalysts [12] , [13] , [14] , [15] , [16] , [17] , [18] . The key to the first strategy is to prepare atomically dispersed metal catalysts, a burgeoning class of catalytic materials, in which isolated metal atoms were anchored on the solid supports [7] , [19] , [20] , [21] , [22] , [23] . Owing to their unique structural and electronic features, the atomically dispersed noble metal catalysts not only displayed unrivaled advantages for their maximal atomic utilization and high turnover frequency (TOF) but also strongly promoted the studies related to active site identifications and reaction mechanisms [23] , [24] , [25] , [26] , [27] , [28] . For the second approach, it is highly desired to develop new catalysts using cheap, non-toxic, and earth-abundant transition metals, such as Cu or Fe, to achieve comparable catalytic performance to that of Pd-based catalysts. Indeed, non-noble metal oxides have been investigated extensively for the development of low-cost and high-performance alkyne hydrogenation catalysts, including ceria [12] , [13] , [14] , [15] , [16] . Owing to limited H 2 activation ability [29] , semihydrogenation of alkynes over these oxide catalysts normally required a relatively high-operating temperature. In an elegant work recently, Pardo et al. reported a metal–organic framework-based Fe(III)-O catalyst [18] . This single-site cationic species was active for acetylene hydrogenation at up to 150 °C, which is an important advance in non-noble metal catalyst for this reaction. Alternatively, earth-abundant metal especially Cu-based catalysts have been developed and evaluated for the reaction, suggesting that Cu, as an inexpensive and non-toxic catalyst, has an activity for acetylene hydrogenation over other aforementioned non-noble metals [30] . Yet, a small quantity of Pd promoter was still a must for achieving satisfactory catalytic performance [31] , [32] . Herein we report the fabrication of cheap atomically dispersed Cu catalysts without other noble metals to effectively catalyze selective hydrogenation of acetylene. In the followings, we will first show adequate experimental evidences that isolated Cu atoms were anchored over the surface-defective nanodiamond–graphene (ND@G) support (Cu 1 /ND@G). Second, we will demonstrate that Cu 1 /ND@G possessed remarkable catalytic performance: high conversion (95%), high selectivity (98%), and good stability (for >60 h) for acetylene hydrogenation, compared to the Cu-cluster catalyst supported over the same host (denoted as Cu n /ND@G). Finally, by density functional theory (DFT) calculations, we will show that the unique structure of the atomically dispersed Cu catalyst facilitates the activation of acetylene and the desorption of ethylene, which is pivotal for the enhanced activity and selectivity of Cu 1 /ND@G compared to Cu n /ND@G. Synthesis and characterization of Cu 1 /ND@G and Cu n /ND@G We prepared the Cu 1 /ND@G and Cu n /ND@G catalysts following the preparation procedure in the “Methods” section. Here we will probe the dispersion states of Cu atoms in these two different catalysts. The substrate ND@G features a thin graphene shell with abundant defects formed during the annealing of ND. High-resolution transmission electron microscope (HRTEM) images (see Fig. 1a and Supplementary Fig. 1 ), Raman spectra, and X-ray photoelectron spectroscopic (XPS) measurements (see Supplementary Figs. 3 and 4 ) revealed the unique defect-rich structure of ND@G. The highly defective few-layer graphene outer-shells served as hosts for anchoring metal atoms. By simply modulating the reduction temperature (see the preparation details in the “Methods” section) of Cu species deposited on graphitic carbon shells, we could change the dispersion state of Cu to prepare two different types of catalysts: atomically dispersed Cu catalyst (denoted as Cu 1 /ND@G) and Cu-cluster catalyst (denoted as Cu n /ND@G). Importantly, both of them have identical Cu loading amount (0.25 wt%). From X-ray diffraction (XRD) profiles (see Supplementary Fig. 5 ), no diffraction associated with bulk Cu was detected on both catalysts, demonstrating that the Cu species were highly dispersed over the substrate surface. 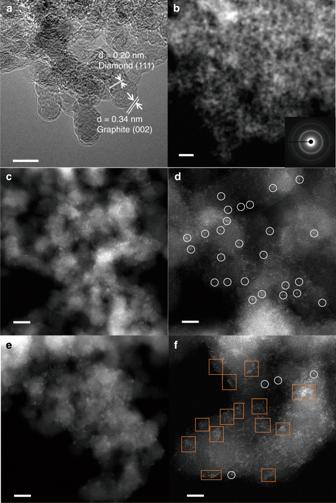Fig. 1 TEM characterization of ND@G support and Cu1/ND@G and Cun/ND@G catalysts.aHRTEM image of ND@G nanocarbon support. Scale bar, 5 nm.bHAADF-STEM image of Cu1/ND@G at low magnification. Scale bar, 20 nm.cHAADF-STEM images of Cu1/ND@G at low magnification. Scale bar, 5 nm.dHAADF-STEM images of Cu1/ND@G at high magnification. Scale bar, 2 nm.eHAADF-STEM images of Cun/ND@G at low magnification. Scale bar, 5 nm.fHAADF-STEM images of Cun/ND@G at high magnification. Scale bar, 2 nm. (The inset attached tobis diamond’s diffraction rings’ image. Atomically dispersed Cu atoms are highlighted by white circles indand Cu clusters are highlighted by orange squares inf.) Further structural analysis of the catalysts (see Supplementary Table 1 ) revealed that no obvious differences in chemical structure were found between Cu 1 /ND@G and Cu n /ND@G except for the dispersion of Cu species. The aberration-corrected high-angle annular dark-field scanning transmission electron microscopic (HAADF-STEM) images showed that the Cu 1 /ND@G catalyst was consisted of isolated bright spots, indicating the atomically dispersed Cu species on ND@G (Fig. 1c, d ). In contrast, for Cu n /ND@G, the Cu species was dominated by Cu clusters, together with a small amount of atomically dispersed Cu (see Fig. 1e, f ). In good agreement with the results of TEM, Cu dispersion state observed by N 2 O titration (99.8% for Cu 1 /ND@G and 85.2% for Cu n /ND@G, see Supplementary Table 1 ) further confirmed that the two catalysts, sharing the same Cu loading, have different atomic dispersion states. Fig. 1 TEM characterization of ND@G support and Cu 1 /ND@G and Cu n /ND@G catalysts. a HRTEM image of ND@G nanocarbon support. Scale bar, 5 nm. b HAADF-STEM image of Cu 1 /ND@G at low magnification. Scale bar, 20 nm. c HAADF-STEM images of Cu 1 /ND@G at low magnification. Scale bar, 5 nm. d HAADF-STEM images of Cu 1 /ND@G at high magnification. Scale bar, 2 nm. e HAADF-STEM images of Cu n /ND@G at low magnification. Scale bar, 5 nm. f HAADF-STEM images of Cu n /ND@G at high magnification. Scale bar, 2 nm. (The inset attached to b is diamond’s diffraction rings’ image. Atomically dispersed Cu atoms are highlighted by white circles in d and Cu clusters are highlighted by orange squares in f .) Full size image The X-ray adsorption fine structure (XAFS) measurement was employed to further investigate the distinct structure of Cu species. Clearly, the near-edge feature of Cu 1 /ND@G or Cu n /ND@G samples was in between of those of Cu foil and CuO (Fig. 2a ), indicating that the Cu species were partially positively charged (Cu δ+ , 0 < δ < 2). Fourier-transformed k 2 -weighted extended X-ray absorption fine structure (EXAFS) in R space was performed to elucidate the coordination environments of Cu atoms anchored on ND@G. For Cu 1 /ND@G, the only distinct scattering was observed at 1.5 Å that corresponds to the first coordination shell of Cu-C or Cu-O. This evidences the single atom Cu on ND@G through Cu-C bonding, which is further verified by the appearance of Cu-C peak at 283 eV in C 1 s XPS spectrum after Cu was loaded on ND@G (Fig. 3a ) [32] . In contrast, for Cu n /ND@G, besides the scattering of Cu-C at 1.5 Å, a major peak at 2.2 Å that ascribed to Cu-Cu scattering could be observed, indicating the formation of Cu clusters. A wavelet transformation (WT) of Cu k -edge EXAFS oscillations also displayed the dispersion of Cu in both samples visually in both k and R spaces. 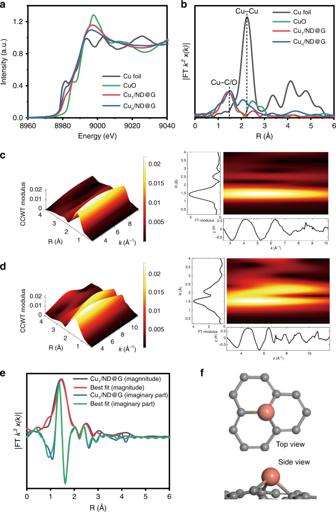Fig. 2 Synchrotron XAFS measurements of Cu1/ND@G and Cun/ND@G catalysts.aCuk-edge XANES profiles for Cu1/ND@G, Cun/ND@G, Cu foil, and CuO.bCuk-edge EXAFS spectra inRspace for Cu1/ND@G, Cun/ND@G, Cu foil, and CuO.cWT analysis of Cu1/ND@G.dWT analysis of Cun/ND@G.eEXAFS fitting curve for Cu1/ND@G.fThe optimized Cu-C3structure; color code: Cu (orange), C (gray) Figure 2c, d are the WT contour plots of Cu 1 /ND@G and Cu n /ND@G that showed a Cu-C back-scattering contribution near 1.5 Å, indicating that both Cu 1 and Cu n were anchored on ND@G through the Cu-C bonding. However, as shown in Fig. 2d , another peak at 2.2 Å in Cu n /ND@G, which is associated with the Cu-Cu scattering, further verified the dispersion state of Cu clusters. Fig. 2 Synchrotron XAFS measurements of Cu 1 /ND@G and Cu n /ND@G catalysts. a Cu k -edge XANES profiles for Cu 1 /ND@G, Cu n /ND@G, Cu foil, and CuO. b Cu k -edge EXAFS spectra in R space for Cu 1 /ND@G, Cu n /ND@G, Cu foil, and CuO. c WT analysis of Cu 1 /ND@G. d WT analysis of Cu n /ND@G. e EXAFS fitting curve for Cu 1 /ND@G. f The optimized Cu-C 3 structure; color code: Cu (orange), C (gray) Full size image Fig. 3 XPS measurements of ND@G support and Cu 1 /ND@G and Cu n /ND@G catalysts. a C 1 s XPS of ND@G, Cu 1 /ND@G, and Cu n /ND@G. b Cu 2 p XPS of Cu 1 /ND@G and Cu n /ND@G Full size image XPS was used to study the valence states of Cu in two catalysts (Fig. 3b ). For Cu 1 /ND@G, the Cu 2 p 3/2 peak appeared at 933.7 eV, situated between Cu 0 /Cu + (932.4 eV) and Cu 2+ (934.6 eV) [33] , [34] , which is consistent with the XANES results (Fig. 2a and Supplementary Fig. 6 ). The results imply that the Cu species in Cu 1 /ND@G interact strongly with the substrate. Through Cu-C bonds, an elevated chemical valence of single atom Cu species due to charge transferred from Cu atoms to substrate could be observed, which was absent on Cu n /ND@G due to the similar properties between Cu clusters and bulk Cu. Quantitative chemical configuration analysis of Cu 1 /ND@G and Cu n /ND@G were carried out through the least-squared EXAFS fitting. The R -space fitting results are shown in Fig. 2e and Supplementary Fig. 9 , and the corresponding structure parameters are listed in Supplementary Table 2 . The coordination number of the center Cu atom with surrounding C atoms on Cu 1 /ND@G was 3.1, and the mean bond length of Cu-C was 1.94 Å. Based on these results, the proposed local atomic structure of Cu was constructed as that in Fig. 2f . The isolated Cu atom was anchored over the defective sites of graphene through bonding with three C atoms. Acetylene hydrogenation performance over Cu 1 /ND@G and Cu n /ND@G Selective hydrogenation of acetylene was carried out using Cu 1 /ND@G and Cu n /ND@G, respectively, to gain insight into the impact of the atomic structure and spatial arrangement of Cu over the catalytic performance. The conversion and selectivity as a function of temperature over these two catalysts are shown in Fig. 4a . For aggregated Cu species in Cu n /ND@G, the conversion was still <20% even at 200 °C. Significantly, Cu 1 /ND@G manifested robust catalytic activity and remarkably high selectivity toward ethylene (see Fig. 4a ). The conversion of acetylene reached 95% at 200 °C, with ethylene selectivity of 98%. We further compared the intrinsic activity of two catalysts, as shown in Fig. 4b . 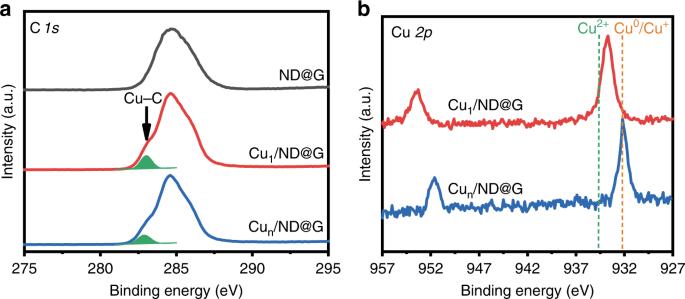Fig. 3 XPS measurements of ND@G support and Cu1/ND@G and Cun/ND@G catalysts.aC 1sXPS of ND@G, Cu1/ND@G, and Cun/ND@G.bCu 2pXPS of Cu1/ND@G and Cun/ND@G Cu 1/ ND@G showed a high TOF of 0.0017 s −1 (4.25 times higher than that of Cu n /ND@G) and a high ethylene yield of 93.1%, showing competitive advantages over former results [<90%] (see Supplementary Table 3 and Supplementary Fig. 10 ). Apparent activation energies ( E a ) of the Cu 1 /ND@G and Cu n /ND@G catalysts were 41.9 and 54.3 kJ/mol, respectively (see Fig. 4c ), suggesting the superiority of atomically dispersed Cu catalysts. The stability of Cu 1 /ND@G catalyst was found to be excellent. As shown in Fig. 4d , the conversion and selectivity at 200 °C over Cu 1 /ND@G remained steady at 95% and 98%, respectively, for at least 60 h under reaction conditions. The atomic structure of the Cu 1 /ND@G catalyst was well maintained (see Supplementary Figs. 7 – 9 and Supplementary Tables 1 and 2 ) during the stability test. Meanwhile, under the reaction conditions where the conversion is high enough to meet the industrialization requirement (see Supplementary Fig. 11 ), Cu 1 /ND@G remained stable for at least 30 h. Fig. 4 Catalytic performance of Cu 1 /ND@G and Cu n /ND@G. a Conversion and selectivity as a function of temperature for the selective hydrogenation of acetylene over the Cu 1 /ND@G and Cu n /ND@G catalysts. b TOF values (in the kinetic region) and ethylene yields ( T = 200 °C) of the catalysts. c Arrhenius plots of the catalysts. d Durability test on Cu 1 /ND@G at 200 °C for 60 h. (reaction condition: 1% C 2 H 2 , 10% H 2 , 20% C 2 H 4 gas mix balanced with He; GHSV = 3000 h −1 ) Full size image DFT calculations To better understand the nature of the superior acetylene hydrogenation activity of Cu 1 /ND@G, the reaction process was studied by DFT. The details of the computational simulation methods can be found in the “Methods” section. Cu 1 supported over graphene layer (Cu 1 @Gr) was used to model the Cu 1 /ND@G catalyst, while a Cu 13 cluster on ND@G to model the Cu n /ND@G catalyst. The computational details are summarized in Supplementary Information , including all of the possible binding modes of different adsorbates on the catalytic surfaces. The energy profiles (including the entropy contribution) for the catalysis of Cu 1 /ND@G are shown in Fig. 5 . 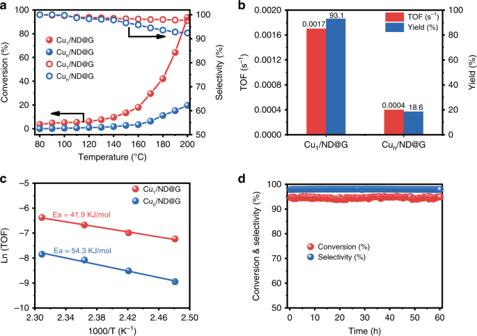Fig. 4 Catalytic performance of Cu1/ND@G and Cun/ND@G.aConversion and selectivity as a function of temperature for the selective hydrogenation of acetylene over the Cu1/ND@G and Cun/ND@G catalysts.bTOF values (in the kinetic region) and ethylene yields (T= 200 °C) of the catalysts.cArrhenius plots of the catalysts.dDurability test on Cu1/ND@G at 200 °C for 60 h. (reaction condition: 1% C2H2, 10% H2, 20% C2H4gas mix balanced with He; GHSV = 3000 h−1) 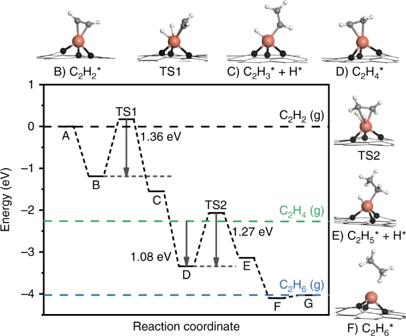Fig. 5 Energy profile of acetylene hydrogenation on the Cu1/ND@G catalyst and the structures of intermediates and transition states. Color code: Cu (orange), C in graphene (black), C in reactant/intermediates/product (gray), and H (white) On Cu 1 /ND@G, the adsorption energy of acetylene on Cu atoms is −1.19 eV (see Supplementary Table 4 ). Then the molecular hydrogen undergoes dissociative adsorption. This step is exothermic by 0.36 eV with an energy barrier of 1.36 eV (from B to C), which is the rate determining step (RDS) for acetylene hydrogenation. On the Cu 13 cluster catalyst, the barrier of RDS is 1.50 eV (see Supplementary Fig. 14 ), implying that the cluster catalyst is less active than the Cu 1 catalyst (see Supplementary Fig. 16 ). More importantly, the transition-state energy of ethylene hydrogenation on Cu 1 /ND@G (TS2, 1.27 eV) is above the energy of gas-phase ethylene (1.08 eV), suggesting that ethylene favors desorption over further hydrogenation in the following step. In another word, the high selectivity of acetylene hydrogenation here is due to the priority of ethylene desorption at the atomically dispersed Cu sites of Cu 1 /ND@G. This calculated result is consistent with the observed difference in catalytic performance between Cu 1 /ND@G and Cu n /ND@G. Fig. 5 Energy profile of acetylene hydrogenation on the Cu 1 /ND@G catalyst and the structures of intermediates and transition states. Color code: Cu (orange), C in graphene (black), C in reactant/intermediates/product (gray), and H (white) Full size image In summary, we synthesized an atomically dispersed Cu 1 /ND@G catalyst for acetylene semihydrogenation reaction. It exhibited remarkably outstanding acetylene conversion (~95%), ethylene selectivity (~98%), and stability (>60 h), exceeding the Cu-cluster catalyst with the same Cu loading. The unique bonding structure and electronic property of Cu atoms on Cu 1 /ND@G facilitate the acetylene activation and ethylene desorption, which clearly elucidates the importance of isolated Cu atoms in catalysts for high-performance acetylene semihydrogenation. Our results and conclusions pave the way for rational design of promising non-noble catalysts for hydrogenation processes. Materials ND powders were purchased from Beijing Grish Hitech Co., Ltd, China. Copper (II) nitrate trihydrate (Cu(NO 3 ) 2 ·3H 2 O) was the analytical reagent and purchased from Sinopharm Chemical Reagent Co., Ltd, China. Deionized (DI) water with the specific resistance of 18.25 MΩ cm was used in all our experiments. Preparation of ND@G ND@G was prepared by annealing ND powders at 1100 °C (heating rate 5 °C min −1 ) for 4 h under flowing Ar gas (100 mL min −1 ) and then naturally cooled to room temperature. The as-prepared products were further purified by hydrochloric acid for 24 h and then washed with DI water. Finally, the ND@G nanocarbon support was obtained after drying in vacuum at 60 °C for 24 h. Preparation of Cu 1 /ND@G and Cu n /ND@G Typically, 200 mg ND@G was dispersed into 30 mL DI water in a 100-mL round-bottom flask, and the mixture was ultrasonically treated for 30 min to obtain a homogeneous suspension. Then the pH value of ND@G support suspension was adjusted to about 11 by dropping 0.25 M Na 2 CO 3 solution. Afterwards, 4 mL Cu(NO 3 ) 2 ·3H 2 O solution (containing 0.125 mg mL −1 Cu) was introduced into ND@G support suspension dropwise under magnetic stirring at 100 °C in oil bath and then kept stirring for 1 h. At the end, the mixture was naturally cooled to room temperature, collected by filter, washed several times with DI water, and dried in vacuum at 60 °C for 12 h. The catalysts were reduced in H 2 (10 vol% in He, flow rate = 50 mL min −1 ) at 200 °C for 1 h to yield Cu 1 /ND@G and at 600 °C for 1 h to obtain Cu n /ND@G. The catalysts after the 60-h reaction were denoted as Cu 1 /ND@G-60h and Cu n /ND@G-60h, respectively. Catalyst characterization methods HRTEM images were taken by a FEI Tecnai G2 F20 working at 200 kV. Atomic resolution STEM images were recorded by a JEOL JEM ARM 200CF aberration-corrected cold field-emission scanning transmission electron microscope at 200 kV. XPS were carried out on ESCALAB 250 instrument with Al Kα X-rays (1489.6 eV, 150 W, 50.0 eV pass energy) and the C 1 s peak at 284.6 eV as internal standard. XRD patterns were collected by using an X-ray diffractometer (Bruker Smart APEX II) using a Cu Kα source at a scan rate of 2° min −1 . N 2 physisorption were measured at −196 °C using a Micrometrics ASAP-2020 instrument. The porosity of samples was obtained through Brunauaer–Emmetr–Teller analysis with the pore volume measured at p / p 0 = 0.99, and the pore size distribution was analyzed by BJH method from desorption branch. The dispersion of Cu species on catalysts was measured by a surface oxidation–reduction method on a AutoChem II 2920 apparatus. Typically, 200 mg sample was loaded in a quartz U-tube. After pretreatment with He at 100 °C for 30 min, the sample was reduced with 10 vol% H 2 in Ar at 200 °C for 1 h (flow rate = 30 mL min −1 ) and cooled to 90 °C in He flow. Then 10 vol% N 2 O in He was introduced into the tube and kept for 3 h at 90 °C (flow rate = 30 mL min −1 ). The sample was purged with He again and cooled to 50 °C, and then the sample was reduced with 10 vol% H 2 in Ar (flow rate = 30 mL min −1 ) from 50 °C to 450 °C with a heating rate of 10 °C min −1 . Ultraviolet-Raman spectroscopy was performed on powder samples by using HORIBA LabRam HR Raman spectrometer, and the excitation wavelength was 325 nm with a power of 0.2 mW (exposure 90 s, accumulate 3 times). XAFS measurements were carried out at Shanghai Synchrotron Radiation Facility. Elemental analysis of copper in the solid catalysts was detected by inductively coupled plasma–atomic emission spectrometry (Optima 8300 DV). Catalytic performance tests The selective hydrogenation activity of the catalysts was conducted in a quartz-bed flow reactor for acetylene hydrogenation with 200 mg catalysts. A gas mixture of 1 vol% C 2 H 2 , 10 vol% H 2 , and 20 vol% C 2 H 4 with He balance (flow rate = 10 mL min −1 , GHSV = 3000 mL g −1 h −1 ) was introduced, followed by ascending temperature testing. Gas chromatograph (GC) injections were done at each temperature after stabilization for 30 min. The reactants and products were analyzed by GC (Agilent 7890 A) equipped with a flame ionization detector and a HP-PLOT AL/S (HP-plot 19091 P-S15, Agilent, 50 m × 0.32 mm × 8 μm) capillary column with He as the carrier gas. Acetylene conversion and selectivity to ethylene were calculated as the following: 
    Conversion = C_2H_2 (feed) - C_2H_2/C_2H_2× 100%
 (1) 
    Selectivity = (1   -  C_2H_6 + 2C_4 olefin/C_2H_2 (feed) - C_2H_2) × 100%
 (2) Computational simulations of the catalytic mechanisms by Cu 1 /ND@G and Cu n /ND@G All of the catalytic structures were obtained by the geometry optimizations using the plane-wave-based DFT method implemented in the Vienna Ab Initio Simulation Package [35] , [36] . We describe the electron–ion interaction using the projector augmented wave method [37] , [38] . The generalized gradient approximation and the Perdew–Burke–Emzerhof functional [39] , [40] describes the exchange and correlation energies for all systems. All the calculations take spin polarized into consideration. The plane-wave expansion of the wave functions adopted an energy cutoff of 400 eV. The Monkhorst–Pack k -point was set to 3 × 3 × 1 in the reciprocal lattice. The convergence criteria for electronic self-consistent interactions is 10 −5 . The geometries of bulk and surface were optimized by the conjugate gradient algorithm until the maximum force on any ion was <0.03 eV Å −1 , where all the atoms in the catalyst and adsorbate were fully relaxed. The most stable configurations of the reactant and intermediates on Cu 1 @Gr were determined by using the climbing image nudged elastic band method [41] , and vibrational frequencies were analyzed to ensure the transition state with only one imaginary frequency.